Proton-coupled sugar transport in the prototypical major facilitator superfamily protein XylE The major facilitator superfamily (MFS) is the largest collection of structurally related membrane proteins that transport a wide array of substrates. The proton-coupled sugar transporter XylE is the first member of the MFS that has been structurally characterized in multiple transporting conformations, including both the outward and inward-facing states. Here we report the crystal structure of XylE in a new inward-facing open conformation, allowing us to visualize the rocker-switch movement of the N-domain against the C-domain during the transport cycle. Using molecular dynamics simulation, and functional transport assays, we describe the movement of XylE that facilitates sugar translocation across a lipid membrane and identify the likely candidate proton-coupling residues as the conserved Asp27 and Arg133. This study addresses the structural basis for proton-coupled substrate transport and release mechanism for the sugar porter family of proteins. The major facilitator superfamily (MFS) of secondary membrane transporters is the largest collection of membrane proteins that are found in all kingdoms of life and includes >15,000 members [1] , [2] . They function as uniporters, antiporters or symporters to catalyse the transport of a wide range of compounds including simple sugars, inositols, drugs, amino acids, oligosaccharides, nucleosides, esters and a large variety of organic and inorganic ions [3] . At least 74 distinct families within the MFS have been identified, and generally each family is responsible for the transport of a single class of compounds [1] . Despite only weak sequence homology, MFS members share a remarkable structural conservation. MFS proteins contain two halves, the N- and C-terminal domains, each formed by a bundle of six or seven transmembrane (TM) helices and the substrate translocation pathway is located at the interface between the N- and C-domains [4] , [5] , [6] , [7] , [8] , [9] , [10] , [11] , [12] , [13] , [14] , [15] , [16] , [17] , [18] , [19] . MFS members were proposed to use an alternating access mechanism for substrate translocation also known as the rocker-switch model [4] , [8] . The transporters can adopt two main open conformations for substrate loading/release, namely the outward- and inward-facing open conformations, and alternate between these two conformations through occluded states to translocate substrates across the membrane [2] . Glucose transporters (GLUTs) are arguably some of the most well-characterized and medically important MFS members. GLUTs belong to the sugar porter [20] family of MFS, whose members are present across all kingdoms of life and are responsible for the transport of sugar across the cellular membrane [3] . In humans, GLUTs are expressed in all cell types where they are primarily responsible for sugar uptake that is then used in metabolic pathways as a primary source of energy [20] , [21] . Diseases such as Type 2 diabetes, hyper- and hypo-glycemia and heart disease typically involve misregulated or mutated GLUTs [20] . Moreover, all known cancers overexpress GLUTs for increased glucose uptake to support uncontrolled cellular proliferation [22] , [23] . Most mammalian GLUT members transport sugars down a concentration gradient by facilitated diffusion in either direction into and out of cells. In bacteria, GLUT homologues such as the Escherichia coli xylose permease (XylE) couple the transport of a H + with the transport of a sugar such as D -xylose against its concentration gradient from the periplasm to the cytoplasm [24] , [25] . XylE is the first member of the MFS that has been structurally characterized in multiple transporting conformations that include both the outward- and inward-facing conformations. Currently, crystal structures of XylE in the outward partially occluded conformation with substrate bound and the inward partially occluded conformations as well as the inward open conformation have been reported, although the latter only at low resolution ( Supplementary Fig. 1 ) [13] , [15] . On the basis of an overlay of these structures, the transition from outward facing to inward facing in XylE was described as a symmetric rigid body movement [26] . However, the dynamics in a lipid membrane and the significance of H + coupling have not been described and remain unclear. Here we report the 3.5 Å resolution crystal structure of XylE in a new inward open conformation, in which the cytoplasmic domain is detached from the TM domain ( Fig. 1 ). We employed molecular dynamic simulations to investigate the transport cycle of XylE in a lipid membrane. Our analysis suggests that in a membrane, XylE functions through a non-symmetric rocker-switch movement. Residues possibly involved in H + coupling are identified, and the role they play in the transport mechanism tested by transport assays following mutagenesis as well as by MD simulations in the protonated and deprotonated state. 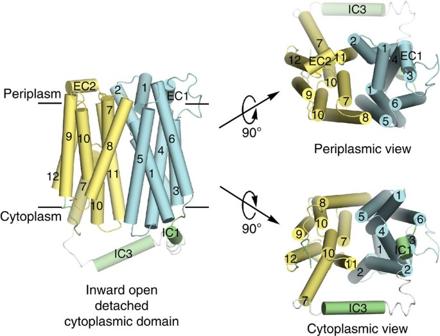Figure 1: Structure of XylE in the inward-facing open conformation with a detached cytoplasmic domain. XylE folds into 12 transmembrane (TM) domains as labelled. TM1-6 form the N-domain (light blue) and TM7-12 form the C-domain (yellow). The substrate translocation pathway is located in between the N- and C-domains. Short helices EC1 and EC2 connect TM3-4 and TM11-12 on the periplasmic side, respectively. A long intracellular linker containing helices IC1–IC3 connects TM6 and TM7. For illustrative purposes, disordered regions in the intracellular linker unobserved in our structure are connected for the figure in white as a reference and were modelled as helices based on the previous crystal structure of XylE (PDB 4GBY). Figure 1: Structure of XylE in the inward-facing open conformation with a detached cytoplasmic domain. XylE folds into 12 transmembrane (TM) domains as labelled. TM1-6 form the N-domain (light blue) and TM7-12 form the C-domain (yellow). The substrate translocation pathway is located in between the N- and C-domains. Short helices EC1 and EC2 connect TM3-4 and TM11-12 on the periplasmic side, respectively. A long intracellular linker containing helices IC1–IC3 connects TM6 and TM7. For illustrative purposes, disordered regions in the intracellular linker unobserved in our structure are connected for the figure in white as a reference and were modelled as helices based on the previous crystal structure of XylE (PDB 4GBY). Full size image Structure of XylE in the new inward-facing open conformation We overexpressed the truncated E. coli XylE (residues 6–480), and purified the protein to homogeneity as described in Methods. Truncated XylE is functional and shows significant accumulation of ( 3 H)- D -xylose above the background in our cell-based uptake assay. Initial crystallization trials yielded narrow hits mainly with polyethylene glycols (PEGs) and zinc acetate as the precipitants. Crystals of XylE formed in the presence of 30 mM D -glucose and a mixture of detergents yielded good data allowing us to solve the structure to 3.5 Å resolution ( Table 1 ). Model building and chain tracing were guided using the structure of XylE in the outward partially occluded conformation (PDB 4GBY) [15] to ensure the fidelity of our model. Regions of the model that deviate from the previous structure were strongly supported by both the omit F o –F c and the 2F o –F c electron density maps ( Fig. 2a,d ; Supplementary Fig. 2a,b ). Our structure was determined from a new crystal form (P3 1 21) and has a much improved resolution over the previously reported structure in the inward open conformation at 4.2–6.0 Å anisotropic resolution [13] , allowing us to identify and describe in detail the conformational change involved in the transport movement. Table 1 Data collection and refinement statistics. 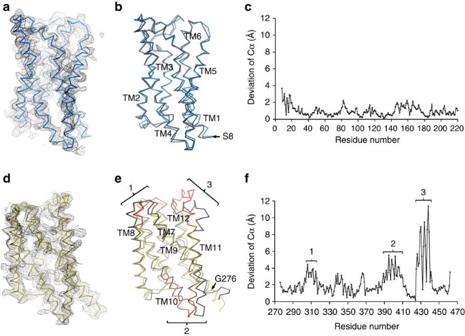Figure 2: Comparison of the N- and C-domains of XylE in the outward-facing partially occluded and the inward-facing open conformations. (a) The Cα backbone of the N-domain from residues 8–220 (light blue) of XylE in the inward-facing conformation looking from the interface between the N- and C-domains. TheσA-weighted 2Fo–Fcelectron density map is displayed here at 1.3σfor clarity. Our density map at 3.5 Å resolution is well defined and allows for accurate determination of positions and conformations of the helices and side chains. (b) Superposition of the N-domain of XylE of the inward-facing conformation with the same domain of the outward-facing conformation (PDB 4GBY). Overall r.m.s.d. of the Cα atoms for the N-domain is 1.1 Å. (c) A corresponding plot of deviation of the Cα positions in the N-domain between the inward- and outward-facing conformations. The N-domain does not appear to undergo a significant conformational change between the two structures. (d) The Cα backbone of the C-domain from residues 270–462 (yellow) of XylE in the inward-facing conformation looking from the interface between the N- and C-domains. TheσA-weighted 2Fo–Fcelectron density map is shown here also at 1.3σ. (e) Superposition of the C-domain of the inward-facing conformation (yellow and red) with the same domain of the outward-facing conformation. Overall r.m.s.d. of the Cα atoms for the residues 276–462 is 2.9 Å. Three regions where the deviations of Cα atoms are higher than 3 Å are highlighted in red. These regions are the helix-loop-helix between TM7-8, TM10-11 and TM11-12, which are the transport interface between the N- and C-domains. Residues 270–275 (not included in the calculation of least square superposition), which are part of the linker in the outward-facing conformation, form a helical extension from the cytoplasmic end of TM7. (f) A corresponding plot of deviation of the Cα positions in the C-domain between the inward- and outward-facing conformations. Regions with large conformational changes (>3 Å r.m.s.d.) ineare indicated. Full size table Figure 2: Comparison of the N- and C-domains of XylE in the outward-facing partially occluded and the inward-facing open conformations. ( a ) The Cα backbone of the N-domain from residues 8–220 (light blue) of XylE in the inward-facing conformation looking from the interface between the N- and C-domains. The σ A -weighted 2F o –F c electron density map is displayed here at 1.3 σ for clarity. Our density map at 3.5 Å resolution is well defined and allows for accurate determination of positions and conformations of the helices and side chains. ( b ) Superposition of the N-domain of XylE of the inward-facing conformation with the same domain of the outward-facing conformation (PDB 4GBY). Overall r.m.s.d. of the Cα atoms for the N-domain is 1.1 Å. ( c ) A corresponding plot of deviation of the Cα positions in the N-domain between the inward- and outward-facing conformations. The N-domain does not appear to undergo a significant conformational change between the two structures. ( d ) The Cα backbone of the C-domain from residues 270–462 (yellow) of XylE in the inward-facing conformation looking from the interface between the N- and C-domains. The σ A -weighted 2F o –F c electron density map is shown here also at 1.3 σ . ( e ) Superposition of the C-domain of the inward-facing conformation (yellow and red) with the same domain of the outward-facing conformation. Overall r.m.s.d. of the Cα atoms for the residues 276–462 is 2.9 Å. Three regions where the deviations of Cα atoms are higher than 3 Å are highlighted in red. These regions are the helix-loop-helix between TM7-8, TM10-11 and TM11-12, which are the transport interface between the N- and C-domains. Residues 270–275 (not included in the calculation of least square superposition), which are part of the linker in the outward-facing conformation, form a helical extension from the cytoplasmic end of TM7. ( f ) A corresponding plot of deviation of the Cα positions in the C-domain between the inward- and outward-facing conformations. Regions with large conformational changes (>3 Å r.m.s.d.) in e are indicated. Full size image The XylE structure contains residues 8–471 forming 12 TM helices divided into two halves, the N- and the C-domains, each containing six TM helices ( Fig. 1 ; Supplementary Fig. 2c ). These two domains are connected through a helical linker (residues 221–275), which is partially disordered in our structure. Two short helices connect TM3-TM4 and TM11-TM12 on the periplasmic side (EC1 and EC2, respectively) (EC2 is disordered in the previous inward-facing structures [13] ). The N- and C-domains of XylE are pseudo-symmetrical and can be superimposed with a root-mean-squared deviation (r.m.s.d.) of 2.8 Å over 155 Cα atoms ( Supplementary Table 1 ). TM1, 2, 7 and 10 show breaks near the center of the helices. Overall, XylE adopts an inward-facing open conformation in our structure. Conformational change based on crystal structure overlays We first compared the individual domains of XylE structures in the outward partially occluded [15] and the inward open conformations. Our analysis revealed that the N-domain (residues 8–220) remained largely unchanged (superposition with r.m.s.d. of 1.1 Å) ( Fig. 2a–c ) while the C-domain (residues 276–462) underwent a significant rearrangement in the transition from an outward to inward-facing conformation (with r.m.s.d. of 2.9 Å) ( Fig. 2d–f ; Supplementary Table 1 ). Helix-loop-helix regions of TM7-TM8, TM10-TM11 and TM11-EC2-TM12 located at the interface between the N- and C-domains show significant conformational deviation of >3 Å of Cα atoms, a result of helical bending ( Fig. 2e,f ). The analysis indicated a non-symmetric conformational change of the two pseudo-symmetrical halves of XylE, in which the N-domain remains mostly rigid while the C-domain is more elastic and undergoes local rearrangements during the transport cycle. This observation is consistent with the analysis of the crystallographic B-factors which are ~40% higher for the C-domain compared with the N-domain. Although the available crystal structures indicate a conformational rigidity in the N-domain, we cannot exclude a possibility that flexibility may occur in the intermediate occluded conformation. As XylE changes its conformation, the interface between the two domains undergoes a significant rearrangement. In the outward partially occluded conformation, the substrate-binding site is partially accessible to the periplasm through a cavity lined by TM1, 2 and 5 from the N-domains, and TM7, 8 and 11 from the C-domains. From the cytoplasmic side, TM10 closes the transporter by interacting with TM4 ( Fig. 3a–c ; Supplementary Fig. 3a,c ). In the inward-facing conformation, all helices in the C-domains move to the same degree with additional conformational change in TM7, 8, 11 and EC2 to completely seal the cavity from the periplasmic side. At the same time, TM10 moves together with the C-domain helices to open up a new solvent-accessible tunnel from the center of the transporter to the cytoplasm ( Fig. 3d–f ; Supplementary Fig. 3b,d ). 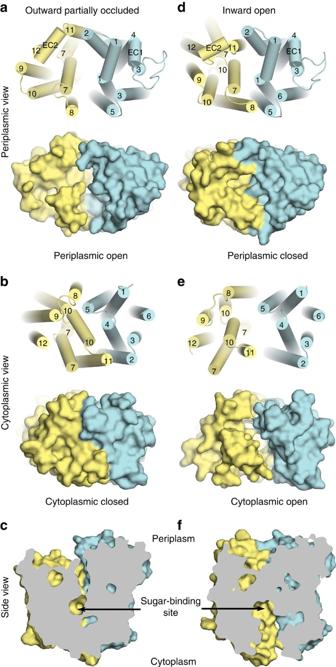Figure 3: Comparison of XylE in the outward-facing partially occluded and the inward-facing open conformation. (a) Periplasmic, (b) cytoplasmic and (c) side views of the outward-facing partially occluded conformation. (d) Periplasmic, (e) cytoplasmic and (f) side views of the inward-facing opened conformation. The N-domain (residues 8–220) is shown in light blue, the C-domain (residues 276–463) in yellow. Cartoon (top) and van der Waals surface (bottom) representations are shown for the periplasmic and cytoplasmic views. Surface cutaway through the sugar-binding site is shown for the side view. The cytoplasmic domain is omitted for clarity. Figure 3: Comparison of XylE in the outward-facing partially occluded and the inward-facing open conformation. ( a ) Periplasmic, ( b ) cytoplasmic and ( c ) side views of the outward-facing partially occluded conformation. ( d ) Periplasmic, ( e ) cytoplasmic and ( f ) side views of the inward-facing opened conformation. The N-domain (residues 8–220) is shown in light blue, the C-domain (residues 276–463) in yellow. Cartoon (top) and van der Waals surface (bottom) representations are shown for the periplasmic and cytoplasmic views. Surface cutaway through the sugar-binding site is shown for the side view. The cytoplasmic domain is omitted for clarity. Full size image The transition from an outward partially occluded to inward open conformation in XylE also includes a large conformational change in the soluble cytoplasmic domain of the protein. In the outward-facing conformation, the intracellular linker between TM6 and TM7 (residues 221–273) folds into three α-helices (referred to as helices IC1–IC3 hereafter) that pack against a short helix from the C terminus (residues 463–479, called helix IC4) [15] . Together IC1-4 form a cytoplasmic soluble four-helix bundle. This bundle caps the substrate translocation pathway in the outward-facing conformation and is stabilized through numerous interactions with TM domains of XylE ( Fig. 4a ). In the inward open conformation, the soluble cytoplasmic bundle of XylE unfolds, becomes partially disordered and swings away from the substrate translocation pathway ( Fig. 4b ). In fact, only part of helix IC1 and IC3 were visible in our electron density map. Likewise, IC4 of the C terminus was disordered and the interactions in the outward-facing conformation appear to be broken. As a result, the cytoplasmic domain shifted away from the substrate translocation pathway by as much as 35 Å. Such a detachment was not observed in previous XylE studies likely because this cytoplasmic domain mediated crystal contacts ( Supplementary Fig. 4a–c ) [13] . In our study, the cytoplasmic domain was not constrained by crystal contacts ( Supplementary Fig. 4d ) and was therefore free to adopt the delocalized conformation effectively exposing the substrate-binding site to the inside of the cell. The new pathway extends well into the very center of XylE from which the substrate could be released. 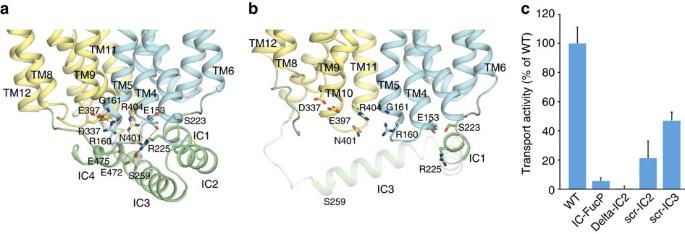Figure 4: Views of the cytoplasmic domain in the outward partially occluded conformation (a) and in the inward open conformation (b). The N-domain is shown in light blue, the C-domain in yellow and the cytoplasmic domain in green. Disordered regions of the intracellular linker are shown in white. Hydrogen bonds and salt-bridges are depicted as grey dashes. (c) Cell-based transport assays of the wild-type full-length XylE and four cytoplasmic domain mutants. For the IC-FucP mutant, the IC2 and IC3 helices were replaced with the intracellular linker of FucP. For the delta-IC2 and scr-IC2 mutants, the IC2 helix sequence was deleted or randomly scrambled, respectively. For the scr-IC3 mutant, the IC3 helix sequence was randomly scrambled. (3H)-D-xylose uptake was normalized to wild type based on protein amount using western blot analysis. Error bars (n⩾5) represent s.e.m. Figure 4: Views of the cytoplasmic domain in the outward partially occluded conformation (a) and in the inward open conformation (b). The N-domain is shown in light blue, the C-domain in yellow and the cytoplasmic domain in green. Disordered regions of the intracellular linker are shown in white. Hydrogen bonds and salt-bridges are depicted as grey dashes. ( c ) Cell-based transport assays of the wild-type full-length XylE and four cytoplasmic domain mutants. For the IC-FucP mutant, the IC2 and IC3 helices were replaced with the intracellular linker of FucP. For the delta-IC2 and scr-IC2 mutants, the IC2 helix sequence was deleted or randomly scrambled, respectively. For the scr-IC3 mutant, the IC3 helix sequence was randomly scrambled. ( 3 H)- D -xylose uptake was normalized to wild type based on protein amount using western blot analysis. Error bars ( n ⩾ 5) represent s.e.m. Full size image To investigate the functional role of the cytoplasmic domain, we generated four XylE mutants in which the helix bundle has been perturbed. The mutants were (i) intracellular helices IC2 and IC3 were replaced with the cytoplasmic linker of the MFS member FucP (IC-FucP) [5] , IC2 helix of XylE was deleted (delta-IC2), (iii) the sequence of the IC2 helix of XylE was scrambled (scr-IC2) and (iv) the sequence of the IC3 helix of XylE was scrambled (scr-IC3). The length of the linker for the IC-FucP mutant was designed to match the distance from end to end of the IC2 and IC3 helices based on structure superimpositions (see Methods for details). In our functional assay, the IC-FucP and delta-IC2 mutants exhibited no significant transport function, while the scr-IC2 and scr-IC3 mutants showed a reduced activity to ~25 and ~50% of the wild type, respectively ( Fig. 4c ). These results indicate that the length and sequence identity of the cytoplasmic domain are important for the transport activity of XylE. The functional and mechanistic role of the cytoplasmic domain in XylE is unclear. There is little sequence conservation in this domain among homologues in this family, which helps explain why our scrambled mutants are still moderately active. We hypothesize that the cytoplasmic domain modulates the transport activity when the transporter switches back from the inward- to the outward-facing conformation by acting as a latch. We speculate that the transport rate would be fast when the cytoplasmic linker IC1–IC3 is intact, as helix IC4 can latch onto the helical bundle effectively. The rate would be slow when the cytoplasmic linker is detached, as IC4 cannot interact with the bundle or the bundle has to first reform. This is consistent with our functional assays that indicate that the uptake is slow when we scrambled the sequence of either the IC2 or IC3 helix to perturb the helical bundle. Interestingly, the cytoplasmic domain of human GLUT1 is also involved in its regulation [27] and a similar latch mechanism was proposed [19] . Conformational transition in a membrane by MD simulations We used targeted molecular dynamics (TMD) simulations [28] to investigate the conformational changes in XylE, as it alternated from the outward- to the inward-facing conformation in the context of a membrane. The transition from the outward partially occluded conformation (with substrate bound) to the inward open conformation is presented in Fig. 5a–c ; Supplementary Fig. 5a,b . We subsequently used steered molecular dynamics (SMD) simulations [29] to study the motion of the sugar molecule exiting the substrate-binding site ( Fig. 5d ; Supplementary Fig. 5c ). The simulations allowed us to visualize a complete translocation of D -xylose through the substrate tunnel in the set 13-ns time scale. For TMD simulations, 1 ns simulation with a small force constant of 0.1 kcal mol −1 Å −2 was sufficient to transform XylE from the outward partially occluded conformation to the inward partially occluded conformation. Moreover, 4 ns simulation was enough to reach the fully opened inward conformation with the same relatively low force constant. However, owing to the highly flexible linker between the N- and C-domains in the cytoplasm, an additional 4 ns simulation was required to reach the target conformation with an increasing force constant stepwise from 0.1 to 0.5 kcal mol −1 Å −2 . Three trials of TMD simulations with different initial velocities provide very similar results, indicating that our TMD data are reproducible and consistent ( Supplementary Fig. 6 ). Therefore, the following data are based on one of the three TMDs. 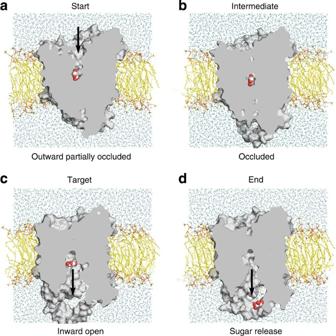Figure 5: Surface cutaway representation of sugar transport pathway from representative molecular dynamics simulation snapshots. (a) The starting outward partially occluded conformation withD-xylose bound, (b) the occluded intermediate, (c) the target inward open conformation and (d) the final sugar release conformation of XylE embedded in the membrane system in the MD simulation box. XylE (van der Waals surface) is embedded in the lipid molecules (yellow and orange lines) surrounded by water molecules (light-blue spheres) and Cl−ions (magenta spheres).D-xylose molecule is shown as white and red large spheres. Figure 5: Surface cutaway representation of sugar transport pathway from representative molecular dynamics simulation snapshots. ( a ) The starting outward partially occluded conformation with D -xylose bound, ( b ) the occluded intermediate, ( c ) the target inward open conformation and ( d ) the final sugar release conformation of XylE embedded in the membrane system in the MD simulation box. XylE (van der Waals surface) is embedded in the lipid molecules (yellow and orange lines) surrounded by water molecules (light-blue spheres) and Cl − ions (magenta spheres). D -xylose molecule is shown as white and red large spheres. Full size image Overall, the motion of XylE in the membrane observed in the MD simulations is different from the movement that was previously reported based on the crystal structure overlays alone [13] , [26] . In our simulations, the periplasmic half of the N-domains showed a significant movement towards the C-domains to close the periplasmic vestibule while the C-domain appeared less mobile. On the cytoplasmic side, however, both the N- and C-domains moved apart with a higher magnitude for the C-domain to open the cytoplasmic vestibule ( Supplementary Fig. 7 ). Sugar release mechanism in XylE In the crystal structure of the outward partially occluded conformation the sugar-binding site in XylE is formed by a number of highly conserved residues. These residues include Gln168 (TM5), Gln288/Gln289/Asn294 (TM7), Trp392 (TM10) and Gln415 (TM11) contributing a total of eight hydrogen bonds with D -xylose. In addition, Phe24 (TM1), Tyr298 (TM7) and Trp416 (TM11) form parts of the sugar-binding pocket ( Figs 3c and 6a ). Mutation of these residues severely diminished XylE function [15] . 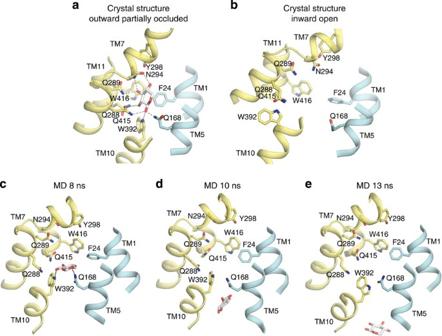Figure 6: Movements in the substrate-binding site for sugar release. (a) Views of the substrate-binding sites of the outward partially occluded conformation and (b) the inward open conformation in the crystal structures of XylE. The N-domain is depicted in light blue and the C-domain in yellow. Hydrogen bonds are depicted as grey dashes. (c–e) Snapshots ofD-xylose translocation in SMD simulations. Figure 6: Movements in the substrate-binding site for sugar release. ( a ) Views of the substrate-binding sites of the outward partially occluded conformation and ( b ) the inward open conformation in the crystal structures of XylE. The N-domain is depicted in light blue and the C-domain in yellow. Hydrogen bonds are depicted as grey dashes. ( c – e ) Snapshots of D -xylose translocation in SMD simulations. Full size image Following the transition to the inward open conformation, most of the residues that form the substrate-binding site shift apart for substrate release in the crystal structure ( Figs 3f and 6b ; Supplementary Fig. 2b ). An exception is Tyr298 in the C-domain above the sugar, which acts as a periplasmic gate to close the substrate-binding site from the periplasm [30] . Trp392 on the other hand acts as a cytoplasmic substrate-release gate. In the outward partially occluded conformation, Trp392 caps the substrate-binding site as it is situated directly underneath the bound sugar and provides a hydrogen bond for sugar coordination. In the inward-facing conformation, Trp392 swings ~6 Å away (measured from Cα atoms) from the adjacent Gln168 in the N-domain opening a tunnel to the center of the transporter and exposing the sugar to the cytoplasm. The long-range movement of the substrate-binding residues completely obliterates the sugar–protein hydrogen bond network, likely resulting in a weaker affinity for sugar and effectively releasing the sugar into the cytoplasm. Consistent with the above, no substrate was observed in the electron density map near the substrate-binding site ( Supplementary Fig. 2b ), although XylE was crystallized with 30 mM D -glucose. MD simulations allowed us to visualize the sugar being translocated from the sugar-binding site towards the cytoplasm. During the TMD simulations, hydrogen bond networks between oxygen atoms of D -xylose and the sugar-binding residues are weakened, as the transporter reorients to the inward open conformation. As a result the sugar appears to flip by ~90° ( Figs 5a–c and 6a versus c ). Gln168 from TM5 and Trp392 from TM10 located near the cytoplasmic side appear to form new hydrogen bonds with the sugar to facilitate its movement towards the cytoplasm ( Fig. 6c ). As the transporter transitions to the inward open conformation, Gln168 and Trp392 move further apart, seemingly to pull the sugar from the center of the protein lower towards the cytoplasm. These MD data are consistent with mutagenesis and functional uptake studies, in which Q168A and W392A mutants showed significantly reduced transport activities [15] . During the subsequent SMD simulations, D -xylose exits the sugar-binding site and continues down along the z axis towards the cytoplasm ( Supplementary Fig. 8 ). At the tunnel exit point, the potential of mean force (PMF) showed a total energy barrier of ~7 kcal mol −1 . This high-energy barrier may correspond to the transient polar and nonpolar interactions between D -xylose and amino-acid residues located in the tunnel ( Supplementary Tables 2 and 3 ; Supplementary Fig. 8c ). Then D -xylose moves downwards and makes brief contacts with the hydrophilic cytoplasmic domain of XylE before it is fully released into the cytoplasm ( Fig. 5d ; Supplementary Video 1 ). The calculated PMF profile from the SMD simulations for pulling D -xylose from the sugar-binding site to the cytoplasm is presented in Supplementary Fig. 8b . Proton-coupled sugar transport Channels and transporters that translocate protons typically have glutamate, aspartate and/or histidine residues that are capable of protonation or deprotonation at the substrate translocation pathway [18] . Structural analysis of XylE reveals two such residues: Asp27 (TM1) and Glu206 (TM6). Sequence analyses of sugar porter members indicate that Asp27 is conserved in homologues that are known to couple the transport of sugar with protons ( Supplementary Fig. 9 ). Mutations of Asp27 in XylE abolished transporter function ( Fig. 7a ). Likewise, mutation of this Asp in other proton-coupled SP homologues also abolished function [9] , [31] , [32] . Mammalian GLUTs, which do not couple the transport of sugar with a proton gradient, contain an asparagine or alanine residue at this position and transport sugar by a facilitated diffusion mechanism. Glu206, on the other hand, is not conserved and the sugar transport activity of XylE was mildly reduced when this residue was mutated ( Fig. 7a ). 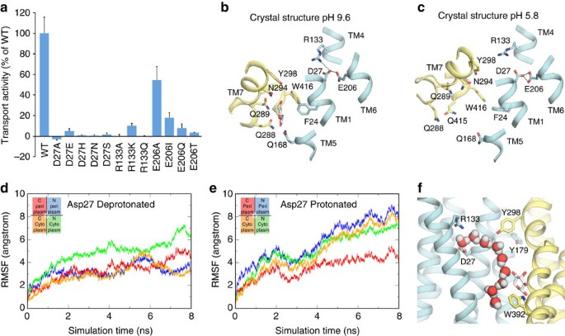Figure 7: Proton -coupled sugar transport. (a) Cell-based transport assays of wild-type full-length XylE as well as D27, R133 and E206 mutants. (3H)-D-xylose uptake was normalized to wild type based on protein amount using western blot analysis. Error bars (n⩾5) represent s.e.m. (b) In the crystal structure of the outward partially occluded conformation at a basic pH, the deprotonated Asp27 interacts with Arg133. (c) In the crystal structure of the inward open conformation at an acidic pH, Asp27 is partially protonated and no longer interacts with Arg133. (d,e) Movements of the backbone of four different subdomains from TMD simulations measured as RMSF from the initial conformation with deprotonated Asp27 indand protonated Asp27 ine. Each subdomain and the corresponding RMSF line are shown with the same colour code: periplasmic N-subdomain (blue); cytoplasmic N-subdomain (green); periplasmic C-subdomain (red); cytoplasmic C-subdomain (orange). Protonation of Asp27 is likely the trigger for the rapid conformational change and substrate release. (f) A possible mechanism for proton release from Asp27 through a water wire trapped inside the solvent cavity of XylE to the cytoplasm. Figure 7: Proton -coupled sugar transport. ( a ) Cell-based transport assays of wild-type full-length XylE as well as D27, R133 and E206 mutants. ( 3 H)- D -xylose uptake was normalized to wild type based on protein amount using western blot analysis. Error bars (n ⩾ 5) represent s.e.m. ( b ) In the crystal structure of the outward partially occluded conformation at a basic pH, the deprotonated Asp27 interacts with Arg133. ( c ) In the crystal structure of the inward open conformation at an acidic pH, Asp27 is partially protonated and no longer interacts with Arg133. ( d , e ) Movements of the backbone of four different subdomains from TMD simulations measured as RMSF from the initial conformation with deprotonated Asp27 in d and protonated Asp27 in e . Each subdomain and the corresponding RMSF line are shown with the same colour code: periplasmic N-subdomain (blue); cytoplasmic N-subdomain (green); periplasmic C-subdomain (red); cytoplasmic C-subdomain (orange). Protonation of Asp27 is likely the trigger for the rapid conformational change and substrate release. ( f ) A possible mechanism for proton release from Asp27 through a water wire trapped inside the solvent cavity of XylE to the cytoplasm. Full size image In the crystal structure of the outward partially occluded conformation of XylE, Asp27 is stabilized by interactions with the conserved Arg133 from TM4 ( Fig. 7b ). Mutation of Arg133 considerably reduced the transport function in XylE ( Fig. 7a ). In addition, naturally occurring mutation of this equivalent residue in human GLUT1 (despite engaging in a non-coupled transport mechanism) was found in patients with GLUT1 deficiency syndrome [33] . Analysis of the XylE structures that were obtained at different pH values suggests that the interaction between Asp27 and Arg133 is affected by the protonation state of Asp27. In the structure of the outward partially occluded conformation obtained at a basic pH of 9.6 with sugar bound, Asp27 is likely deprotonated (predicted pKa of ~4.6 by the H++ server [34] from the structure) and stabilized by interactions with Arg133 ( Fig. 7b ). Asp27 also interacts with a non-conserved Glu206 residue from TM6, which is solvent inaccessible and always protonated (predicted pKa of ~12). Because Asp27 is distant from the sugar-binding site and XylE can bind sugars even at a basic pH, it is likely that sugar binding is proton independent. In the structure of the inward open conformation obtained at an acidic pH of 5.8, Asp27 no longer interacted with Arg133 but maintained the interaction with Glu206 ( Fig. 7c ). Prediction of pKa by the H++ server [34] suggested that Asp27 in this conformation has a pKa of 5.2, and is likely partially protonated at the crystallization pH. We hypothesize that protonation of Asp27 breaks the interactions with Arg133 and could act as a trigger for switching XylE from the outward- to inward-facing conformation to translocate sugar to the cytoplasm. However, how the interactions between Asp27 and Arg133 affect the transport is unclear and cannot be explained by the crystal structures alone. To further investigate the functional role of Asp27 and Arg133 in proton-coupling transport, TMD simulations with different protonation states of Asp27 were calculated. Deprotonated Asp27 maintained salt bridge and hydrogen bond interactions with Arg133, and Glu206 throughout the entire 8 ns TMD simulations ( Fig. 8a,c ). In sharp contrast, protonated Asp27 showed significantly higher degree of freedom and broke the hydrogen bond interactions with Arg133 and Glu206 during the simulations ( Fig. 8b,d ). Overall, the transport dynamics were significantly altered with different Asp27 protonation states. 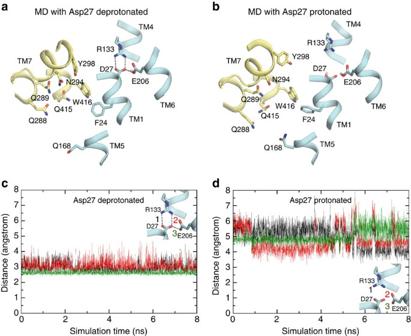Figure 8: Interactions of Asp27 at different protonation states in MD simulations. (a,b) Snapshots of MD trajectory representing interactions of Asp27 in TM1 with Arg133 and Glu206 from neighbouring helices (TM4 and TM6). (a) When Asp27 is deprotonated, it maintains interaction with Arg133 and Glu206. (b) When Asp27 is protonated, the interactions between Asp27 and Arg133 are broken. At neutral pH, E206 is protonated and neutral while R133 is protonated (proton not shown) and positively charged in all of our simulations based on the H++ pKa prediction. (c,d) Distances from Asp27 to Arg133 (O–N atoms) (black and red lines) and Asp27 to Glu206 (O–O atoms) (green line) during the course of MD simulation. When Asp27 deprotonated, ~3 Å interactions are maintained throughoutc. When Asp27 is protonated, these interactions are broken as the distances between these atoms increase to 4–6 Å (d). Distance between each atom pair is colour coded as shown in the inset inc. Figure 8: Interactions of Asp27 at different protonation states in MD simulations. ( a , b ) Snapshots of MD trajectory representing interactions of Asp27 in TM1 with Arg133 and Glu206 from neighbouring helices (TM4 and TM6). ( a ) When Asp27 is deprotonated, it maintains interaction with Arg133 and Glu206. ( b ) When Asp27 is protonated, the interactions between Asp27 and Arg133 are broken. At neutral pH, E206 is protonated and neutral while R133 is protonated (proton not shown) and positively charged in all of our simulations based on the H++ pKa prediction. ( c , d ) Distances from Asp27 to Arg133 (O–N atoms) (black and red lines) and Asp27 to Glu206 (O–O atoms) (green line) during the course of MD simulation. When Asp27 deprotonated, ~3 Å interactions are maintained throughout c . When Asp27 is protonated, these interactions are broken as the distances between these atoms increase to 4–6 Å ( d ). Distance between each atom pair is colour coded as shown in the inset in c . Full size image To visualize the effect of protonation on the transport cycle of XylE, we analysed the movement of protein versus time in the two TMD simulations (one where Asp 27 was deprotonated and one in which it was protonated). In our analysis, we arbitrarily divided the initial structure into four equal parts by the xy -plane and the yz -plane centering at the bound sugar (periplasmic N- (blue), cytoplasmic N- (green), periplasmic C- (red) and cytoplasmic C-subdomains (orange)). The movement of each subdomain from the initial structure were measured as root-mean-squared flexibility values of the backbone Cα atoms over the course of 8 ns TMD simulation without structural alignment, and plotted against simulation time ( Fig. 7d,e ). (The calculations did not include the motions of the linker between the N- and C-domains in the cytoplasm.). The analysis indicates that the protonation state of Asp27 affected the dynamics of XylE. The periplasmic N-subdomain and the cytoplasmic C-subdomain move significantly more when Asp27 is protonated than when Asp27 is deprotonated. However, the protonation state of Asp27 did not appear to affect the periplasmic C-subdomain and the cytoplasmic N-subdomain. Because TMD simulations use external force addition for each Cα atom to steer a large conformational change to the target direction in a short time scale, the conformational change observed in the trajectories of the deprotonated Asp27 model could be a result from a forced transition to the target. Nevertheless, since the same force constant and the same simulation setup was used in both simulations and yet different dynamics were observed, one must conclude that the differences are important. We propose that when Asp27 is deprotonated, it forms tight interactions with Arg133 and Glu206 in the periplasmic N-subdomain, which could suppress the conformational change of XylE, possibly resulting in a slow transport rate. The protonation of Asp27 possibly weakens these interactions and accelerates the transition from outward- to inward-facing conformations to translocate the substrate to the cytoplasm more efficiently. We further propose that without a proton gradient across the membrane from the periplasm to the cytoplasm, the tight interactions within deprotonated Asp27, Arg133 and Glu206 possibly slow down the conformational change and the transport rate. This is consistent with previous biochemical experiments showing that XylE transports sugar at significantly lower rates in the absence of a proton gradient [26] . Future kinetic experiments will be required to test this hypothesis. It is likely that water is co-transported with the sugar in XylE. Indeed, several water molecules were observed in our simulations in the sugar-binding site, and a solvent-filled cavity connecting Asp27–Arg133 site to the sugar-binding site was observed in the crystal structures of both the inward- and outward-facing conformations of XylE [15] . Moreover, water permeability has been documented for human GLUT members of the SP family [35] , [36] , [37] , [38] . We present a new inward-facing open conformation of the prototypical MFS protein, the H + /xylose symporter XylE. This transporter has been captured in a number of conformational states that include the outward and inward open states. Mutational, functional as well as molecular dynamic simulations allow us to propose a detailed mechanism for sugar transport through this MFS member. The conformational change from outward to inward facing involved an asymmetric movement of the two halves of the transporter with respect to one another. During this transition, the location and orientation of residues important for substrate binding in the substrate-binding site change to either allow the substrate to bind or for substrate release. The proton is likely transported through the charged residue pair Asp27–Arg133. Our MD simulations indicated that XylE transports water molecules along with the substrate. When XylE was transitioning to the inward-facing conformation, water molecules in the tunnel were disconnected from bulk water on the periplasmic side by hydrophobic residues, including Tyr179 and Tyr298. Interestingly, we observed a hydrogen bond network among water molecules in the solvent cavity that formed a water wire connecting the protonated Asp27 and bulk water in the cytoplasm when XylE reached the inward-facing conformation ( Fig. 7f ). This water wire was stable during the course of the final 2 ns of TMD simulations with sugar bound and was broken soon after the sugar was released in SMD simulations. We propose that once the conformational change is complete and the substrate-binding site is open to the cytoplasm, the proton could be transferred through the water wire and released to the cytoplasm before the release of sugar. On the basis of our analysis, we propose that the transport mechanism proceeds in a stepwise manner: The protonation of Asp27 and the binding of sugar to the substrate-binding site together may trigger and accelerate the conformational change in the transporter to switch from the outward- to the inward-facing conformation. The opening of the substrate-binding site to the cytoplasm allows a proton from Asp27 to be transferred through the water wire in the solvent cavity and released into the cytoplasm. The conformational change also assists the sugar movement along the transport pathway for the sugar to exit to the cytoplasm. After both the proton and the sugar have dissociated to the cytoplasm, the interaction between Asp27 and Arg133 could then be re-established and may help accelerate XylE to transition back to the outward-facing conformation to complete the transport cycle. It is possible that a similar mechanism is manifested in some other MFS members helping explain their remarkable characteristics of high affinity for substrates and high efficiency of transport. Protein expression and purification Truncated, wild-type XylE (residues 6–480) gene was PCR amplified from the genomic DNA of the E. coli strain BL21(DE3). The gene was subcloned into pET-15b vector (EMD Millipore) and transformed into E. coli strain BL21 C43(DE3). The E. coli containing the XylE expression plasmid was cultured in Luria-Bertani (LB) media at 37 °C and 250 r.p.m. The cultures were shifted to 18 °C when OD 600 reached 0.5, and the expression of XylE was induced by the addition of 0.5 mM Isopropyl β-D-thiogalactopyranoside (IPTG). The overnight cultures were harvested by centrifugation at 3,000 g and cell pellets were collected and resuspended in 25 mM Tris HCl pH 8 and 150 mM NaCl. A Microfluidizer M110-P processor (Microfluidics Corp) was used for cell lysis at 20,000 psi. The lysate was centrifuged at 10,000 g for 30 min at 4 °C. The supernatant was collected and centrifuged at 150,000 g for 1 h at 4 °C. The membrane pellets were resuspended in 25 mM Tris HCl pH 8 and 150 mM NaCl. XylE was solubilized from the membrane by addition of 5% w/v decyl-β- D -maltopyranoside (Affymetrix) in 10 mM Tris HCl pH 7.5 to a final concentration of 1% w/v. The mixture was rotated at 4 °C for 2 h, then centrifuged at 150,000 g for 45 min at 4 °C. The supernatant was incubated with Ni-NTA resins (Qiagen) in the presence of 25 mM imidazole. The resins were washed with 25 and 50 mM imidazole, respectively, in 10 mM Tris HCl pH 7.5, 150 mM NaCl and 0.2% w/v DM, and XylE was subsequently eluted with 300 mM imidazole in the same buffer. The His-tag was cleaved off overnight at 4 °C using 1 unit of human α-thrombin (Enzyme Research Laboratories) per 1 mg of XylE and 2.5 mM CaCl 2 . XylE was subsequently screened for detergents by size-exclusion chromatography on a Superdex S200 column in 10 mM Tris HCl pH 7.5, 150 mM NaCl with various detergents. XylE was concentrated to ~5–6 mg ml −1 for crystallization. Crystallization XylE crystals were initially obtained in the presence of DM or dodecyl-β- D -maltopyranoside under a broad range of PEG and zinc acetate. However, after extensive optimization the crystals only diffracted poorly to ~8–10 Å resolution. Crystals were significantly improved upon an exchange of detergent into 10 mM Tris HCl pH 7.5, 150 mM NaCl, 0.1% w/v nonyl-β- D -glucopyranoside (NG) and 0.005% w/v decyl maltose neopentyl glycol (Affymetrix) on the Superdex S200 column. XylE in the nonyl-β- D -glucopyranoside/decyl maltose neopentyl glycol mixed detergents was concentrated to 6 mg ml −1 and flash frozen in liquid nitrogen. D -glucose was added to XylE at 30 mM final concentration and the protein was crystallized with 7–12% w/v PEG 8,000, 0.1 M MES pH 5.6–6.0 and 0.1 M zinc acetate, to the size of ~50 μm. Crystals were coated with polyphenyl ether (Santovac-5 cryo oil) (Hampton Research) for cryo-protection and subsequently frozen under liquid nitrogen before data collection. Data processing and structure determination X-ray diffraction was collected at the Stanford Synchrotron Radiation Lightsource (SSRL) beamline 12-2 at 1.127 Å to measure anomalous scattering from zinc near its absorption edge. The diffraction data were indexed and integrated using the program Mosflm [39] , [40] , scaled and merged using the program Aimless/Scala [41] and converted to amplitudes using the program Truncate [41] , [42] in space group P3 1 21. Data statistics from Aimless suggested anisotropic diffraction with mean ( I / σI ) >2.0 at 3.2 Å along l axis and 3.88 Å overall. However, using the half-data set correlation criterion [43] , the data have CC 1/2 >0.5 at 3.5 Å in all directions. Therefore the data were processed to 3.5 Å resolution. The XylE structure was solved by molecular replacement (MR) with the program Phaser [44] using the XylE N-terminal TM domain (residues 5–220) of the outward-facing conformation as a search model (PDB 4GBY) [15] , which gave a clear solution. No MR solution was found using the C-terminal TM domain (residues 275–463). The density map from MR clearly shows the location of helices in the C-terminal TM domain that differ from the previously published XylE structure in the outward-facing conformation. The use of ellipsoidal truncation (at 4.0 Å in the h and k direction, and 3.5 Å in the l direction where mean ( F / σF ) >3) and anisotropy scaling of the data generated by the anisotropy server ( http://services.mbi.ucla.edu/anisoscale ) significantly improved the quality of the density map. Twining analysis, using the program Xtriage in the Phenix crystallography program suite [45] suggested a twinned data set. Therefore, the anisotropy truncated data were used throughout the refinement process with -h , -k , l twin law during the twinned refinement in the program Phenix [45] , which decreased the initial refinement R free from >50% in the non-twinned refinement to ~45%. To facilitate model building in the C-domain, the high-resolution structure of XylE [15] was used as a guide to accurately trace amino-acid registers in the protein chain. Cycles of model building were carried out manually in the program Coot [46] , followed by refinement in Phenix. Helix-loop-helix regions in the C-domain at the transport interface, namely TM7-8, TM10-11 and TM11-12 ( Fig. 2e,f ) show significant deviations in their Cα atoms from the previous structure in the outward-facing conformation [15] . These differences are strongly supported by the 2F o –F c electron density map. When these regions are removed from the C-domain structure of the outward-facing conformation, a clear MR solution was found right away for the C-domain, emphasizing the major differences between the two structures. The location of residues in the MR model solution agrees with our structure and the electron density from MR phases for the excluded region confirms the accuracy of our chain tracing. After the refinement R free dropped below 35%, the model was thoroughly inspected by omitting every 10 residues and rebuilt based on the F o –F c and the 2F o –F c omit electron density maps to reduce model bias in the N-domain from MR and the possible model inaccuracy in the C-domain carried over from the poor initial MR phases. Cycles of refinement were carried out until model completion with refinement twin fraction=0.1, R work =30.8%, R free =32.4% and good geometry ( Table 1 ). The asymmetric unit contains one molecule of XylE from residues 8 to 471 (with disordered residues 229–246 and 262–268) with one zinc ion (as judged by a 5 σ peak in the anomalous difference map) coordinating His158 and possibly unresolved residues in the N terminus. Two XylE monomers pack against one another in an anti-parallel fashion in the crystal with their twofold symmetry (parallel to the membrane plane) coincides with the crystallographic twofold symmetry. Sequence alignment Sequence alignment of XylE and representatives of sugar porter [20] family members were obtained from UniProt ( www.uniprot.org ). The list of homologues are as follows with Uniprot accession number in parentheses: Escherichia coli XylE (P0AGF4); Lactobacillus brevis D -xylose/H + symporter XylT (O52733); Escherichia coli galactose permease GalP (P0AEP1); Escherichia coli arabinose permease AraE (P0AE24); Bacillus subtilis myo-inositol/H + transporter IolT (O34718); Arabidopsis thaliana inositol/H + symporter INT1 (Q8VZR6); Arabidopsis thaliana hexose/H + symporter STP1 (P23586); Parachlorella kessleri hexose/H + symporter HUP1 (P15686); Homo sapiens facilitated glucose transporter GLUT12 (Q8TD20); Homo sapiens H + /myo-inositol transporter GLUT13 (HMIT) (Q96QE2); Homo sapiens facilitated glucose transporter GLUT2 (P11168); Homo sapiens facilitated glucose transporter GLUT10 (O95528); Homo sapiens facilitated glucose transporter GLUT1 (P11166); Homo sapiens facilitated glucose transporter GLUT3 (P11169); Homo sapiens facilitated glucose transporter GLUT4 (P14672); Homo sapiens facilitated glucose transporter GLUT5 (P22732); Homo sapiens facilitated glucose transporter GLUT6 (Q9UGQ3); Homo sapiens facilitated glucose transporter GLUT7 (Q6PXP3); Homo sapiens facilitated glucose transporter GLUT8 (Q9NY64); Homo sapiens facilitated glucose transporter GLUT11 (Q9BYW1); Homo sapiens facilitated glucose transporter GLUT14 (Q8TDB8). Simulation system setup The crystal of structure of XylE with substrate bound in the outward-facing partially occluded conformation (PDB 4GBY) was used as initial coordinates. The pKa values of titratable residues were calculated with the H++ server ( http://biophysics.cs.vt.edu/H++ ), a computational prediction system for the pKa values of ionizable groups in macromolecules based on the Poisson–Boltzman (PB) or generalized Born (GB) models [34] . The protonation states of each residue were assigned based on the pKa calculations at pH 7. The protein was incorporated perpendicularly into a 100 × 100 Å POPC bilayer in the xy -plane. Overlapping lipids were removed and TIP3P water molecules [47] were filed along the z axis with 15 Cl − counterions to neutralize the system in a 100 × 100 × 98 Å box. All water molecules and xylose found in the X-ray crystal structure were included. The RESP charges of POPC [48] , [49] and D -xylose were derived using RED version 3 [50] , [51] . For introducing the protonated state of Asp27, the same system was constructed with one additional hydrogen atom on Asp27 and one Cl − ion to provide a neutral environment. Conventional molecular dynamics simulations With initial configurations with or without protonation of Asp27, the waters, ions, sugar and lipids in the box were initially minimized by 5,000 steps of steepest descent minimization followed by another 2,500 steps of conjugated gradient minimization, keeping the protein constrained to their initial position. Thereafter, the entire system was minimized without restraints by the same protocol. A 2-ns relaxation simulation was performed with imposing restraint energy potential of 20 kcal mol −1 for all of the peptide atoms. All bonds involving hydrogen atoms were constrained using the SHAKE algorithm. A nonbonded cutoff distance of 12 Å and a time step of 2 fs were used. Then, a 20-ns simulation was performed with the same protocol without restraints ( Supplementary Fig. 5d,e ). All MD simulations were carried out using the AMBER package (version 11) employing ff99SB force field combined with GAFF force field [52] , [53] at constant temperature (300 K), constant pressure (1 atm) and periodic boundary conditions. Two snapshots at 3 and 20 ns were used as input structures for further TMD simulations. TMD simulations Three trials of 8 ns TMD simulations (one starting from the 3-ns equilibration snapshot and two from the 20-ns equilibration snapshot of the previous conventional MD simulations of the outward-facing conformation) with or without a protonation of Asp27 were performed with random seed numbers. The crystal structure of the inward-facing open conformation from this study was used as the target structure (PDB 4QIQ ). Owing to the disordered parts in the crystal structure, the Cα atoms of residues 9–226, 248–260 and 269–470 were restrained to the corresponding atomic positions of the target structure to force the conformation change. The targeted RMSD value to the final structure was 1.0 Å. A force constant of 0.1 kcal·mol −1 Å −2 was sufficient for the protein to open inwards over 4 ns, and the force was subsequently increased stepwise from 0.2 kcal·mol −1 Å −2 to 0.5 kcal·mol −1 Å −2 for the last 4 ns to reach the closest target structure. SMD simulations SMD simulation was employed to pull down the sugar through the tunnel from the inward-facing fully opened conformations obtained from the previous TMDs. Ten independent simulations were calculated using random seeds. The distance between the O5 atom of D -xylose and the CG atom of Leu260 in the cytoplasmic linker between the N- and C-domain of XylE was gradually decreased with a constant rate of 3.5 Å ns −1 without a specific direction. This pulling speed has been shown to be slow enough for sampling [54] . To prevent drifting during the pulling process, the Cα atoms of residues 418 and 179 located far away from the binding pocket and Leu260 were restrained with the harmonic potential of 20 and 100 kcal mol −1 , respectively. The PMF was estimated based on the Jarzynski’s equality <exp[− W / k B T ]>=exp[−Δ G / k B T ], where W is the total nonreversible work done on the system, Δ G is the free energy change between the initial and final states, T is temperature and k B is the Boltzmann constant [55] , [56] , [57] . In addition, the linear extrapolation and the cumulative integral extrapolation methods [58] were used for constructing the PMF from SMDs. For each extrapolation method, the calculation was repeated 500 times to obtain an average and s.d. of PMF. A per-residue decomposition of the sugar-binding free energy was performed using MMPBSA (Molecular Mechanics-Poisson Boltzmann Surface Area) [59] , [60] to evaluate a contribution from each residue during a sugar release. MMPBSA computes the binding free energy by a thermodynamic cycle as a sum of the gas-phase energies, solvent free energies and entropic contributions averaged over snapshots of the MD simulation. Nonpolar solvation energy terms were calculated using a generalized Born (GB) model [59] , [60] . Mutagenesis of XylE Full-length wild-type XylE (residues 1–491) gene was PCR amplified from the genomic DNA of E. coli strain BL21(DE3) and subcloned into pET-15b vector (EMD Millipore). Point mutations of full-length XylE were generated using the QuickChange Lightning site-directed mutagenesis protocol (Agilent Technologies). The XylE cytoplasmic domain mutations were generated based on the PCR-driven overlap extension protocol [61] using Phusion DNA polymerase (Thermo Scientific). Nucleotides corresponding to residues 232–267 of helices IC2 and IC3 were replaced with nucleotides corresponding to cytoplasmic linker E. coli FucP (residues 237–256) to generate the IC-FucP mutant. The length of the linker was carefully chosen based on superposition analysis of crystal structures of FucP (PDB 3O7Q) [5] to match a required distance between end points of the replaced IC2 and IC3 region in XylE in both the outward- and inward-facing conformations. Nucleotides corresponding to residues 232–244 of helix IC2 were deleted to create the IC2 deletion mutant (delta-IC2). To generate the IC2 sequence scramble mutant (scr-IC2), amino-acid residues 232–244 (KQEQAEGILRKIM) were randomly scrambled to the following sequence: ELGIIQKMREKQA. For the IC3 sequence scramble mutant (scr-IC3), amino-acid residues 246–266 (NTLATQAVQEIKHSLDHGRKT) were randomly scrambled to the following sequence: TDTHAQLAELTVGSIKHRKQN. Cell-based uptake assay Uptake of ( 3 H)- D -Xylose was measured using a modified protocol from [62] . E. coli strain BL21(DE3) transformed with pET-15b vectors containing full-length wild-type XylE, truncated XylE as used for crystallization, mutations of full-length XylE or no insert were grown overnight in LB medium, diluted 1:100 in fresh medium and grown to an OD 600 of ~1.0–1.5 at 37 °C. Leaky expression from the pET-15b vector provided sufficient protein expression for the assay as judged by western blot and no specific inducer was added to overexpress the protein. The cells were harvested by centrifugation, washed with ice-cold buffer containing 10 mM MOPS pH 7.3 and 10 mM magnesium sulphate and resuspended in the same buffer to a final OD 600 of 25. ( 3 H)- D -xylose in 90% ethanol (American Radiolabeled Chemicals) containing 5 pCi total radiation was added to 500-μl aliquots of cells and allowed to incubate at room temperature for 1 min. The final concentration of D -xylose in the uptake assay mixtures was 50–100 μM. The cells were collected by rapid filtration, washed with 20 ml of buffer and the filters submitted for liquid scintillation counting. Uptake was normalized based on western blots and protein amounts. Our measurements are close to the initial rate of transport, where the transport K M =63–169 μM based on a previous study [63] . All figures in this paper were prepared with Pymol version 1.5 and assembled in Photoshop CS6 (Adobe). The movie was created in VMD [64] . All plots were generated by Grace ( http://plasma-gate.weizmann.ac.il/Grace/ ). How to cite this article: Wisedchaisri, G. et al . Proton-coupled sugar transport in the prototypical major facilitator superfamily protein XylE. Nat. Commun. 5:4521 doi: 10.1038/ncomms5521 (2014). Accession codes : The atomic coordinates and structure factors have been deposited in the Protein Data Bank with the accession number 4QIQ .